Attomolar DNA detection with chiral nanorod assemblies Nanoscale plasmonic assemblies display exceptionally strong chiral optical activity. So far, their structural design was primarily driven by challenges related to metamaterials whose practical applications are remote. Here we demonstrate that gold nanorods assembled by the polymerase chain reaction into DNA-bridged chiral systems have promising analytical applications. The chiroplasmonic activity of side-by-side assembled patterns is attributed to a 7–9 degree twist between the nanorod axes. This results in a strong polarization rotation that matches theoretical expectations. The amplitude of the bisignate ‘wave’ in the circular dichroism spectra of side-by-side assemblies demonstrates excellent linearity with the amount of target DNA. The limit of detection for DNA using side-by-side assemblies is as low as 3.7 aM. This chiroplasmonic method may be particularly useful for biological analytes larger than 2–5 nm which are difficult to detect by methods based on plasmon coupling and ‘hot spots’. Circular polarization increases for inter-nanorod gaps between 2 and 20 nm when plasmonic coupling rapidly decreases. Reaching the attomolar limit of detection for simple and reliable bioanalysis of oligonucleotides may have a crucial role in DNA biomarker detection for early diagnostics of different diseases, forensics and environmental monitoring. Chirality of nanoparticles (NPs) and their assemblies have recently attracted substantial interest among materials scientists [1] , [2] , [3] , [4] , [5] . There now exist examples of NP assemblies with pyramidal [3] , [6] , [7] and helical morphologies [2] , [8] , and strong chiral responses are predicted for other geometries [9] , [10] . The chiro-optical properties of nanomaterials originate from the atomic-scale chirality of the inorganic core of NPs [11] , the chiral arrangement of the thiolates on their surfaces [12] , the electronic ‘imprint’ of chirality due to adsorbed chiral organic molecules on NPs surface (for example, DNA and peptides) [13] , [14] , and from the intrinsic chiral geometry of NPs or their assemblies at nano- and submicron-scales [2] , [3] , [6] , [7] , [8] . Currently, chiral nanostructures are prepared using chiral templates, for instance, DNA including the origami approach [2] , helical fibres [15] , twisted nanoribbons [8] or by lithography [16] , and the primary motivation for the development of chiral nanomaterials is the possibility of creating chiral metamaterials with negative refractive indices [17] . Optical devices utilizing these phenomena are intriguing, but fundamental challenges remain for the practically relevant infrared and visible range. In this study, we pursue the bioanalytical potential of self-assembled chiral nanoscale superstructures. We demonstrate that the limit of DNA detection reached by side-by-side (SBS) assemblies of Au nanorods (NRs) using chiral bisignate plasmonic signals could be markedly lower than those reported for other widely discussed optical methods employing ultraviolet–visible absorption [18] of coupled plasmons, fluorescence tagging [19] and surface-enhanced Raman scattering (SERS) [20] . In addition, these results compete well for single molecular detection of analytes [21] , due to an alternative dependence of optical polarization effects between interdistant plasmonic particles. NR assemblies by PCR In this study, chiral assemblies of gold NRs were made using a polymerase chain reaction (PCR) ( Fig. 1a ) [22] . The use of PCR allowed for the controlled growth of NP and NR assemblies connected by DNA, where the number of thermal cycles determined the lengths and complexity of the resulting superstructures ( Fig. 1 ). The mode of attachment of NRs to each other followed either an end-to-end (ETE) or a SBS assembly pattern, controlled by the placement of the PCR primers ( Fig. 1 ). 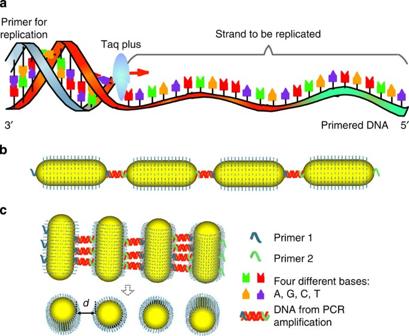Figure 1: Schematics for PCR assembly of Au NRs. (a) PCR replication procedure in which a DNA strand can be ampilified using primer, template DNA, taq plus polymerase and four different DNA bases. (b) PCR-based gold NRs ETE assembly. (c) PCR-based gold NRs SBS assembly with inter-NR gapd; in the bottom part of the panel the DNA chains were removed for clarity. Figure 1: Schematics for PCR assembly of Au NRs. ( a ) PCR replication procedure in which a DNA strand can be ampilified using primer, template DNA, taq plus polymerase and four different DNA bases. ( b ) PCR-based gold NRs ETE assembly. ( c ) PCR-based gold NRs SBS assembly with inter-NR gap d ; in the bottom part of the panel the DNA chains were removed for clarity. Full size image The gold NRs had lengths and diameters of 62 nm and 22 nm, respectively, with an aspect ratio of 2.9. Preferential binding of thiol-terminated primers to the end facets of the NRs allowed for the ETE growth mode for the NR chains ( Fig. 1b ) [5] . To obtain SBS assemblies, Au NRs were modified by dithiothreitol (DTT) binding to the end sites and thiol polyethylene glycol. These modifications make NRs stable for a wide range of solution conditions and protects them from excessive modification by thiols [22] . Subsequent addition of the thiolated primer resulted in preferential attachment to the sides of the NRs. Once introduced to the PCR replication system, NRs modified with DNA strands either at their sides or ends acted as ‘monomers’ for the PCR assembly ( Fig. 1c ) and ‘building blocks’ for the resulting nanoscale assemblies. Variations in the placement of the primers allowed for finely controlled synthesis of extended NR ‘chains’ and ‘ladders’. The number of PCR cycles, n , regulated the length of the assemblies ( Figs 2a–f and 3a–f , Supplementary Figs S1–S11 ). The NR attachment patterns were retained until n =20 and 30 for ETE and SBS assemblies, respectively ( Supplementary Figs S6, S11 ). Modified Au NRs without PCR ( n =0) organized sporadically ( Figs 2a and 3a ). The consistent elongation of NR ‘chains’ and ‘ladders’ with increasing n was confirmed by dynamic light scattering measurements of the hydrodynamic diameter ( D h ). For the ETE assembly, D h increased from 102±2.1 to 701±15 nm as n increased from 2 to 20 cycles. For the same values of n , D h increased from 88±3.1 to 408±23.2 nm in the case of SBS assembly ( Supplementary Fig. S12 ). This change in D h correlates well with the increase of statistically averaged number of NRs in ETE and SBS assemblies for different n values ( Supplementary Figs S13–S17 ). As expected, the length of ETE is greater than those for SBS assemblies because of the sideway attachment of NRs in the latter case. In concert with previous studies [23] , the transverse plasmon for the ETE assembly changed very little with n ( Fig. 2 ), whereas the longitudinal peak shifted to the red ( Fig. 2g ). For the SBS assemblies ( Fig. 3a–f ), the longitudinal plasmon band ( λ L ) experienced a blue shift by 17 nm from n= 0 to n = 30 ( Fig. 3i,k ). 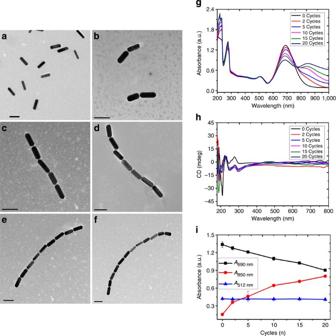Figure 2: Structure and optical properties of ETE assemblies of Au NRs. (a–f) Representative TEM images for ETE assembly obtained after different number of PCR cycles,n=0 (a), 2 (b), 5 (c), 10 (d),15 (e) and 20 (f); scale bar, 50 nm. (g,h) Ultraviolet–visible (g) and CD spectra (h) for ETE assembly obtained for differentn. (i) Intensity of absorption maxima for ETE assemblies obtained for differentn. The error bars represent the standard deviation of sample measurements. Figure 2: Structure and optical properties of ETE assemblies of Au NRs. ( a – f ) Representative TEM images for ETE assembly obtained after different number of PCR cycles, n= 0 ( a ), 2 ( b ), 5 ( c ), 10 ( d ),15 ( e ) and 20 ( f ); scale bar, 50 nm. ( g , h ) Ultraviolet–visible ( g ) and CD spectra ( h ) for ETE assembly obtained for different n . ( i ) Intensity of absorption maxima for ETE assemblies obtained for different n . The error bars represent the standard deviation of sample measurements. 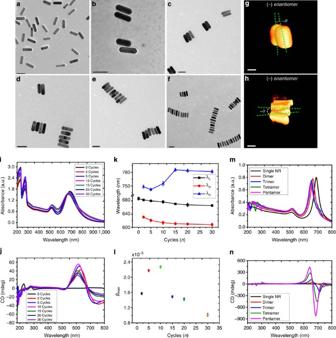Figure 3: Structure and optical properties of SBS assemblies of Au NRs. (a–f) Representative TEM images for SBS assemblies obtained after different number of PCR cycles,n=0 (a), 2 (b,c), 5 (d), 10 (e) and 15 (f); scale bar, 50 nm. (g,h) Cryo TEM tomography images for NRs SBS assembled trimer (g) and pentamer (h); scale bar, 25 nm. (i,j) Experimental ultraviolet–visible (i) and CD spectra (j) for SBS assemblies withn=0–30. (k) Evolution of spectral features of SBS NR assemblies represented byλL(longitudinal peak maximum in ultraviolet–visible spectra),λp(positive peak in plasmonic part of the CD spectra) andλn(negative peak in plasmonic part of the CD spectra) with increasingn. (l) Dependence of the maximum of chiral anisotropy factorgmaxonn. (m,n) Calculated absorption (m) and CD spectra (n) for NRs SBS assemblies. The number of NRs,n,ranged from 1 to 5. The error bars iniandlrepresent the standard deviation of sample measurements. Full size image Figure 3: Structure and optical properties of SBS assemblies of Au NRs. ( a – f ) Representative TEM images for SBS assemblies obtained after different number of PCR cycles, n= 0 ( a ), 2 ( b , c ), 5 ( d ), 10 ( e ) and 15 ( f ); scale bar, 50 nm. ( g , h ) Cryo TEM tomography images for NRs SBS assembled trimer ( g ) and pentamer ( h ); scale bar, 25 nm. ( i , j ) Experimental ultraviolet–visible ( i ) and CD spectra ( j ) for SBS assemblies with n= 0–30. ( k ) Evolution of spectral features of SBS NR assemblies represented by λ L (longitudinal peak maximum in ultraviolet–visible spectra), λ p (positive peak in plasmonic part of the CD spectra) and λ n (negative peak in plasmonic part of the CD spectra) with increasing n . ( l ) Dependence of the maximum of chiral anisotropy factor g max on n . ( m , n ) Calculated absorption ( m ) and CD spectra ( n ) for NRs SBS assemblies. The number of NRs, n, ranged from 1 to 5. The error bars in i and l represent the standard deviation of sample measurements. Full size image Chiral properties of the NR assemblies The chiroptical properties of the NR assemblies and evaluation of their prospects for bioanalysis were the primary foci of this work. A distinct CD signal was seen in the ultraviolet part of the spectrum from 180 to 250 nm for both ETE and SBS assemblies. This should be attributed to DNA ligands and is expected for this system. A strong bisignate CD wave was seen in the plasmonic λ L part of the spectrum between 500 and 800 nm. For the Cotton effect, the 620–800 nm spectral window was negative, whereas for 500–620 nm wavelengths it was positive, which has definitive analogies in molecular systems [24] although displaying greater CD intensity and g- factors ( Fig. 3g , Supplementary Fig. S18 ). Chirality of the assemblies was observed only for SBS and not for ETE assemblies or single DNA-modified NRs ( Figs 2h and 3j ). The strong chiroplasmonic response was observed for n as few as two ( Fig. 3j ) when assemblies of 2–4 NRs were dominant ( Supplementary Fig. S14a ). We saw progressively stronger CD signals as n increased, indicating that chiral geometries of NR assemblies persisted along with increasing the length of SBS assemblies. Appearance of the CD signal should be attributed to the twisted structure of the SBS assemblies [22] . The three-dimensional (3D) images of the assemblies obtained with state-of-the-art cryo transmission electron microscopy (TEM) tomography showed a distinct and consistent twist between two adjacent NRs in the SBS assemblies ( Fig. 3g,h ) [22] . Note these images reflect the conformation of the assemblies as they exist in solution and are not affected by high-vacuum conditions and drying. The negative values of the dihedral angle ( θ ) between the adjacent NRs in SBS assemblies corresponding to the right rotating enantiomers ( Supplementary Fig. S16 ) persist throughout the PCR assembly process [22] . These dihedral angles for dimer, trimer, tetramer and pentamer were consistently negative and equal to −9.0, −7.1, −8.0 and −7.0 degrees, respectively ( Fig. 3g,h , Supplementary Figs S16, S17 ). The preference for one enantiomer as opposed to another is related to symmetry breaking of the parallel NR due to twisting of the connected DNA bridges and the general preference of non-parallel orientation of charged nanoscale rods as the conformation with minimal energy with multiple examples in biomolecules [22] . The consistency of the sign of θ leads to strong chirality of SBS-assembled NRs. ETE assemblies do not exhibit CD response ( Fig. 2h ) because the torsional force of chiral DNA oligomers connecting one end of the rod to another is substantially smaller than in SBS assemblies and therefore the enantiomer distribution is equilibrated. Chirality of the twisted NR assemblies was predicted theoretically [10] but was never observed experimentally [5] until recently [22] . Unlike earlier studies by Kadowala and coworkers on chiroplasmonic shifts on chiral coatings [25] , the prospects for analytical and other applications of their chiroplasmonic properties of twisted assemblies in solutions were not considered theoretically or experimentally. We hypothesized it to be a promising research direction due to the intensity of the chiral signals in these assemblies, their bisignate nature, stronger polarization rotation in solution than in thin films and continuous increase of the CD signal for 0< n<10. The peak values of the anisotropy factor ( g -factor) increased from 1.6 × 10 −3 to 2.3 × 10 −3 with 2–10 cycles ( Fig. 3l , Supplementary Fig. S18 ). As the number of PCR cycles increased, both positive ( λ p ) and negative ( λ n ) CD bands exhibited spectral shifts. The λ p CD band moved to the blue part of the spectrum by 24 nm as PCR cycles increased from 2 to 20 cycles ( Fig. 3k ), whereas λ n shifted by 16 nm from 2 to 5 cycles and became broader after 5 cycles. Also important is that as n exceeds a certain threshold value, the amount of disorder increases and the CD intensity of the bands stops growing. The larger aggregates do not have the consistency in the signs of their dihedral angles and therefore their CD signals decrease ( Fig. 3i ). For n =20, complex agglomerates formed ( Supplementary Fig. S11 ) and racemization of the assemblies occurred. The absorbance ( Fig. 3n ) and CD ( Fig. 3m ) spectra calculated for SBS assemblies of 2–5 NRs showed excellent agreement with experimental results. The simulated electric fields on gold surface ( E -fields) under right/left circular polarized (RCP/LCP) light excitation at λ p and λ n bands showed that the twisted SBS assemblies were indeed chiral: the coupling efficiencies to RCP and LCP ( Supplementary Fig. S19 ) differ considerably. Agreeing with experimental results, the ETE-assembled structure did not show any CD signal ( Fig. 2h ) in the plasmonic region. The simulations of ETE NR trimer performed according to the 3D geometry-based state-of-the-art cryo TEM tomography and indeed exhibited a very weak CD signal ( Supplementary Fig. S20 ). NR assemblies for attomolar DNA biosensing Chirality of SBS assemblies employing different reactant DNA templates can be potentially used for biosensing of oligonucleotides. The possibility of improving the limit of detection (LOD) by taking advantage of the bisignate wave-shape of the CD signals can be one of the advantages of the method. As n increases, λ p becomes more positive, whereas λ n becomes more negative. These spectroscopic changes occur in synch with each other, which essentially increases the detected signal and improves the signal-to-noise ratio. Note also that nanoscale assemblies amplify the chiral adsorption compared with the atomic-scale chirality in organic molecules. In addition to amplification of signal due to bisignate nature of the CD wave and nanoscale dimentions of chiral chromophores, there are also other factors related to dependence of intensity of CD signal on inter-NR gap, d . This dependence is conducive to ultrasensitive detection of biomacromolecules and represents one of the key advantages of this methods compared to others based on plasmon coupling. We evaluated CD and other spectral optical responses for different amounts of target DNA oligomers. The calculated LOD was found to be 3.9 aM, 8.1 aM and 3.7 aM based on CD intensity of C( λ p ), C( λ n ) and C( λ p )–C( λ n ), respectively ( Fig. 4 ). The LOD values above characterizes this techniques as substantially more sensitive than typical PCR methods with or without NPs that give LOD=0.1 fM (ref. 26 ). To validate the bioanalysis by chiroplasmonic effects, the widely used dilution method (see Methods) with a priori known concentrations of DNA was adopted ( Supplementary Fig. S21 ). The concentrations returned by the chiroplasmonic method matched those expected for the specific dilution. The uncertainty coefficient, u , was as low as 0.0367 (see Methods) and indicative of the high accuracy of the method. Such u is associated, among other factors, With PCR amplification, high g , and improved signal-to-noise ratio due to bisignate nature of the chiroplasmonic spectra. 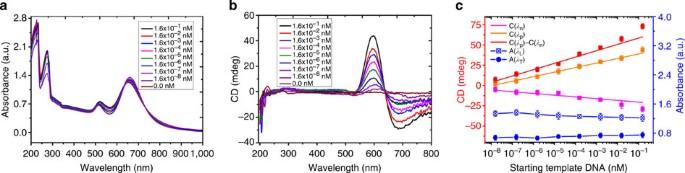Figure 4: DNA analysis with SBS NRs assemblies. (a,b) Experimental ultraviolet–visible (a) and CD spectra (b) for NR assemblies obtained for different DNA concentrations starting from 0.156 nM with stepwise 10 × dilution. (c) Calibration curves obtained using CD and ultraviolet–visible spectra of SBS assemblies. The error bars represent the standard deviation of sample measurements. Figure 4: DNA analysis with SBS NRs assemblies. ( a , b ) Experimental ultraviolet–visible ( a ) and CD spectra ( b ) for NR assemblies obtained for different DNA concentrations starting from 0.156 nM with stepwise 10 × dilution. ( c ) Calibration curves obtained using CD and ultraviolet–visible spectra of SBS assemblies. The error bars represent the standard deviation of sample measurements. Full size image The use of CD spectroscopy is not uncommon for biosensing and sometimes offer better levels of detection compared with ultraviolet–visible [18] , fluorescence spectroscopy [27] , and electrochemistry-based methods [28] , with the best LODs equal to 10,200 and 500 fM, respectively, especially in combination with plasmonic substrates [29] , [30] . However it never reached the level of attomolar (10 −18 M) level of detection. The femtomolar detection level (10 −15 M) is not sufficient to meet the demands of biomedical and environmental applications for a variety of clinical tasks especially for reliable early diagnosis of diseases using DNA biomarkers in complex biological samples. It is relevant to compare analytical capabilities of chiroplasmonic method with its parent/related techniques, for instance, PCR and SERS that do not use CD spectra modulated by plasmonic particles. In some cases methods based on polaron coupling were able to reach nearly single-molecule detection capabilities [20] and high clinical relevance for detection of prostate cancer [21] . We compared chiroplasmonic method with well-established and highly sensitive reverse transcription PCR (RT-PCR) used for clinical and forensic purposes. LOD for the same DNA strands as in Fig. 4 was found to be 156 aM for RT-PCR ( Supplementary Fig. S22 ). The NR assembly method was, therefore, ca. 40 times more sensitive than RT-PCR. The parallel experiments with chiroplasmonic method yielded identical concentrations with the chiroplasmonic bioanalysis. Analytical capabilities of SERS are being rapidly advanced in many laboratories including successful SERS analysis using ETE and SBS assemblies of Au NRs [23] , [31] featuring high-intensity E -fields between the rods, and therefore, deserve special attention in this study. One of the best case scenarios for DNA detection would probably be the use a high-intensity SERS tag, such as 4-aminothiophenol (4-ATP) with Raman-active transitions υ (C–S) at 1,083 cm −1 and υ (C–C) at 1,590 cm −1 . Its SERS signal is further enhanced by E- fields on gold surface amplified after bridging of NRs by DNA. The Raman intensity of 4-ATP increased with increasing n for ETE assemblies with addition of new NRs ( Fig. 5a , Supplementary Figs S23–S25 ). Note that Lee et al. [31] observed a continuous decrease of SERS and E- field intensity with increasing numbers of NRs in SBS assemblies, whereas CD signal in DNA-bridged ETE assemblies display the opposite trend and increase for n< 10 which contributes to improved sensitivity of the chiroplasmonic method. LOD using the strongest SERS line of 4-ATP at 1,083 cm −1 was 1.14 and 1.58 fM for SBS and ETE assemblies ( Fig. 5b ), respectively, which is 290 and 403 times higher than for chiroplasmonic method for the identical DNA strand. Importantly, detection of long DNA is inherently suboptimal using SERS because formation of hotspots critical for its success requires the gaps between NRs to be small, that is, ca. 0.5–2 nm. The same is also true for SERS detection of all high molecular weight compounds that are larger than the size of optimal hotspots and similar spectroscopic methods based on strong polaron coupling, such as surface-enhanced Raman optical activity [24] . Molecules with diameters >2 nm are particularly common in bioanalysis. As indicated by the calculations in Fig. 5c,d , the read-out parameter used in chiroplasmonic method, C( λ p )–C( λ n ), is much less sensitive to the distance between the NRs than the surface E -field necessary to enhance scattering from 4-ATP or other Raman tags. In fact, it initially increases for DNA-relevant size regime rather than decreasing as E- field intensity. Polarization rotation reaches maximum for the NR gap of ca. 20 nm, whereas the intensity of the surface E- field generated by NRs drops off dramatically when gap reaches 5 nm ( Fig. 5c , Supplementary Fig. S26 ). 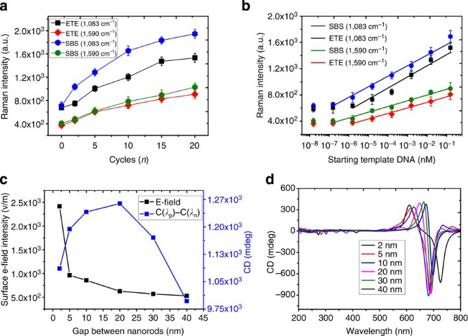Figure 5: DNA analysis using SERS capabilities. (a,b) SERS intensity of 4-ATP tag at 1,083 cm−1and 1,590 cm−1for ETE and SBS NR assemblies obtained after differentn(a) and different starting DNA concentrations (b). (c) Calculated dependence of the intensity of the surfaceE-field and CD intensity for a NR pentamers with gaps of 2, 5, 10, 20, 30 and 40 nm. (d) Calculated CD spectra for NR pentamers with gaps of 2, 5, 10, 20, 30 and 40 nm. The error bars represent the standard deviation of sample measurements. Figure 5: DNA analysis using SERS capabilities. ( a , b ) SERS intensity of 4-ATP tag at 1,083 cm −1 and 1,590 cm −1 for ETE and SBS NR assemblies obtained after different n ( a ) and different starting DNA concentrations ( b ). ( c ) Calculated dependence of the intensity of the surface E -field and CD intensity for a NR pentamers with gaps of 2, 5, 10, 20, 30 and 40 nm. ( d ) Calculated CD spectra for NR pentamers with gaps of 2, 5, 10, 20, 30 and 40 nm. The error bars represent the standard deviation of sample measurements. Full size image We showed that the SBS assemblies of plasmonic NRs with strong polarization rotation make possible detection of DNA markers with unusually low LOD that is greatly needed for medical diagnostics, forensics and environmental needs. The physical phenomena behind this capability include enhancement of polarization rotation by plasmonic structures, chiral symmetry breaking for SBS assemblies and bisignate nature of CD spectra. Chiroplasmonic method of detection has sensitivity advantage for the analysis of biomolecules >2 nm, while other plasmonic methods could be preferred for smaller analytes, unless steps for narrowing the gap by depositing additional layers of plasmonic material are taken. In perspective, the high sensitivity of the CD signal to geometry of the twisted NR assembly allows for experimental observation of the torsional dynamics of helical systems in solutions and better understanding of the 3D geometry of plasmonic assemblies.The strong polarization rotation in DNA-bridged SBS assemblies can also be utilized in intracellular monitoring of low-occurrence markers and signaling molecules. [39] Au nanorod preparation Au NRs were synthesized by Au seeds growth method [32] . Synthesis of Au seeds: hydrogen tetrachloroaurate trihydrate (HAuCl 4 ·3H 2 O) was dissolved in 2.5 ml, 0.2 M hexadecyltrimethylammonium bromide (CTAB) solution, added by 0.3 ml pre-cooled 300 μl, 0.01 M sodium borohydride (NaBH 4 ) and quickly mixed for 2 min and left to reaction at 25 °C for 2 h. The growth of Au NR, 0.15 ml of 0.004 M AgNO 3 (NR): 70 μl of 0.079 M (ascorbic acid, Vc) was added to 5 ml, 0.001 M, HAuCl 4 was added to 5 ml, 0.2 M CTAB solution and left to reduce for 2 min, finally 12 μl of prepared Au seeds were added, strongly stirred for 20 s and left at 25 °C. The concentration of gold NRs was 0.25 nM. NR modification Modification of Au NRs included primer on end, side and 4-ATP modifications. End modification A 1 ml aliquot of synthesized Au NRs was first centrifuged (10,000 g , 10 min). The precipitate was then dissolved in 200 μl of 0.005 M CTAB solution (five times concentrated). The Au NRs modification of the primer was carried out at 25 °C for 12 h with a reaction ratio of 80:1 between the Au NRs and the primer. Then unreacted primer was removed by centrifuging (7,000 g , 10 min) and dissolved in 200 μl of 0.005 M CTAB solution. Side modification A 1 ml aliquot of synthesized Au NRs was five times concentrated into 200 μl of 0.005 M CTAB solution by centrifugation. Then the end sites were modified with DTT for 8 h with a molar ratio of 10:1 between the Au NRs and the primer. The DTT-modified Au NRs were centrifuged again (7,000 g , 10 min) and dissolved in 200 μl of 0.005 M CTAB solution. Then the Au NRs were modified by the addition of polyethylene glycol with a molar ratio of 120:1. Finally, the side modification of the primer was reacted for 10 h at a molar ratio of 400:1 between the primers and the Au NRs. The Au NRs were then centrifuged (70,000 g , 10 min) and stored in 200 μl of 0.005 M CTAB solution. SERS tag modification For SERS measurement, 4-ATP was used to modify the Au NR after being modified by primers. The 4-ATP was modified after the primer was attached with the same modification ratio for end and side modifications. Generally, 4-ATP modification employed similar procedures with the same reaction ratio as that of the NRs modified with primer. The molar ratio between the Au NRs and the 4-ATP was set at 400:1 and reacted for 8 h both for the NRs used for ETE and SBS assemblies. The Au NRs were then centrifuged at 70,000 r.p.m. for 10 min and finally dispersed in 200 μl of 0.005 M CTAB solution. After 4-ATP modification, the as-prepared NRs were employed in PCR-based assemblies with different cycles and the assembled products were monitored in the liquid phase. PCR conditions and Au NR assembly Using Lambda DNA as a template [23] , the PCR reaction was performed in a 100 μl amplification system. The reaction mixture contained 10 μl of PCR buffer, 2 μl of dNTPs (1 mM), 1 μl of template DNA, 1 μl (5 U) of Taq Plus polymerase and 10 μl of each Au NR-forward/reverse-primer (F/R-primer) conjugates (Au NR-F/R-primer); finally, amplification mixture was set to 100 μl by adding 66 μl of ultrapure water. The 5 × PCR buffer contained of 50 M KCl, 10 mM tris–HCl, pH 9.0 at 25 °C, 0.1% TritonX-100 and 1.5 mM MgCl 2 . Each of the Au NR-F/R-primer conjugates and Au NR-reverse-primer (R-primer) conjugates were concentrated to 1.25 nmol. The thermal cycling protocol began with a 3 min predenaturation step at 94 °C, followed by varying cycles of 94 °C denaturation (30 s), 60 °C annealing (30 s) and 72 °C extension (1 min) steps, followed by a further extension for 10 min at 72 °C. Last, the PCR system was held at 4 °C for ca. 10 min before use. Sequences for F-primer and R-primer were listed as follows: F-primer: TGGCTGACCCTGATGAGTTCG; R-primer: GGGCCATGATTACGCCAGTT. The assembly parameter of PCR cycle ( n ) and starting template DNA was set as follows: the n was set as 0, 2, 5, 10, 15, 20 and 30 cycles with starting template DNA concentration of 0.156 nM. The template DNA concentration was set by 10 times stepwise dilution of the starting material, 0.156 nM to 0.0156, fM. Analytical calculations, experimental statistics and uncertainty analysis The LOD was calculated according to the high sensitivity analysis. The calibration curve was plotted as where a and b are the variable obtained via least-square root linear regression for the signal–concentration curve for variable y representing the CD signal (mdeg) at DNA concentration of x (nM). When where s.d. is the standard deviation and C blank is the CD of signal of blank sample (without DNA). The LOD was calculated as follows: The uncertainty for LOD of our assay was calculated using statistical analysis methods based on standard deviations of different concentration points (A-type uncertainty). The standard deviation (s.d.) was calculated according to the well-known formula: where n r is the total number of the samples. X i is the i th sample of the series of measurements. X avg is the average value of the CD (or other) signals obtained for the specific series of identical samples repeated n r times. The uncertainty coefficient, u was calculated as follows: The sample repeat number, n r , was n r =9 for all of the experiments. For DNA detection following the chiroplasmonic protocol presented below, the uncertainty coefficient was 0.0367. According to the methods of uncertainty analysis accepted in analytical chemistry [33] , this value of uncertainty coefficient corresponds to a high accuracy method. Calibration protocol Progressive dilution method with known concentrations of analytes is used for calibration of a wide variety of analytical methods including those for exceptionally small concentrations and single-molecule detection limits. These methods can be based on ultraviolet–visible [18] , fluorescence spectroscopy [27] , or electrochemistry [28] . The reliability of this calibration technique stems from the high accuracy of volume measurements when a sample of known (high) concentration is diluted according to the power law. The template DNA concentrations was acquired by stepwise 10 × dilution, following the procedure accepted in the field of bioanalysis and other branches of analytical chemistry [18] , [34] . For each dilution, 5 μl DNA solution (by pipette with 1–10 μl measurement range) was added to 45 μl (by pipette with 5–50 μl measurement range) ultra-pure water. The pipette tips were replaced and discarded every time. Analogous procedure was carried out for the blank experiment without starting DNA analyte and was used in equation (2) as C blank . One microlitre of as-diluted DNA solution for a specific concentration was added into 100 μl PCR system for amplification and subsequent analysis by CD spectroscopy. RT-PCR detection protocol The RT-PCR was performed by standard procedure according to the process described by Ma et al. [35] RT-PCR was carried out on CFX-96 real-time PCR system with 25 ml amplification volume. The PCR amplification mixture was composed of 1.5 ml 20 × EvaGreen dye, 2.5 ml of 1 mM dNTP, 2.5 ml of 10 × PCR buffer, 0.25 ml of 5 U Taq DNA polymerase and 0.5 ml of 2.5 mM upstream and downstream primer, respectively, and finally ultra-pure water was added to have a volume of 25 ml. The PCR cycling parameters were set as 94 °C denaturation (30 s), 60 °C annealing (30 s) and 72 °C extension (1 min) steps, followed by a further extension for 10 min at 72 °C. Fluorescence measurements were taken after each annealing step. The standard curve for RT-PCR is plotted in Supplementary Fig. S22 according to the number of the threshold cycle, n threshold , defined as the number of PCR cycles when the fluorescence reached the value of 900 (a.u.) for specific concentration of DNA (exponential amplification stage). Computer simulations Computer simulations ETE and SBS assemblies were performed using CST Microwave Studio [36] , [37] . The geometry of the NR ladders and chains was defined by d , surface-to-surface gap between Au NRs, the angle between the long axes of the two NRs. The propagation of excitation beam was defined by φ x and φ z , the angles between excitation beam and x axis, z axis, respectively. The surface of gold NR is composed of two semispherical surfaces and one side cylinder surface. Surface E -field simulations by RCP and LCP were carried out at λ p and λ n, respectively. Surface E -field enhancement simulations were carried out using linearly polarized beam with E -field vector parallel and perpendicular with longitudinal direction of NR. The total E -field enhancement was the sum of these two fields. Simulations of CD and absorbance spectra were accomplished by parameter sweep of φ z and φ x from 0 to 2 π with step of π/ 6 (30°), which was similar to theoretical methods previously explored [9] , [14] , [38] . Instrumentation The ultraviolet–visible spectra were measured using a ultraviolet–visible spectrometer (200–1,000 nm) in a quartz cell. The CD spectra were performed on a Bio-Logic MOS-450 CD spectrometer. TEM micrographs were collected on a JEOL-2010 microscope operated at 120 kV. The 3D reconstruction of electron tomography was carried out using a Tecnai Spirit 120 kV TEM. Dynamic light scattering data were obtained using a Malvern Zetasizer ZS instrument with a 632.8 nm laser source and a backscattering detector at 173°. Raman scattering spectra were measured in liquid cell using a LabRam-HR800 Micro-Raman spectrometer with Lab-spec 5.0 software. The slit and pinhole were set at 100 and 400 mm, respectively, an air-cooled He-Ne laser for 632.8 nm excitation with a power of ~8 mW. How to cite this article: Ma, W. et al. Attomolar DNA detection with chiral nanorod assemblies. Nat. Commun. 4:2689 doi: 10.1038/ncomms3689 (2013).